Microbial biosynthesis of the anticoagulant precursor 4-hydroxycoumarin 4-Hydroxycoumarin (4HC) type anticoagulants (for example, warfarin) are known to have a significant role in the treatment of thromboembolic diseases—a leading cause of patient morbidity and mortality worldwide. 4HC serves as an immediate precursor of these synthetic anticoagulants. Although 4HC was initially identified as a naturally occurring product, its biosynthesis has not been fully elucidated. Here we present the design, validation, in vitro diagnosis and optimization of an artificial biosynthetic mechanism leading to the microbial biosynthesis of 4HC. Remarkably, function-based enzyme bioprospecting leads to the identification of a characteristic FabH-like quinolone synthase from Pseudomonas aeruginosa with high efficiency on the 4HC-forming reaction, which promotes the high-level de novo biosynthesis of 4HC in Escherichia coli (~500 mg l −1 in shake flasks) and further in situ semisynthesis of warfarin. This work has the potential to be scaled-up for microbial production of 4HC and opens up the possibility of biosynthesizing diverse coumarin molecules with pharmaceutical importance. Thromboembolic diseases, including venous thromboembolism and arterial thrombosis, are a leading cause of patient morbidity and mortality worldwide. Annually, venous thromboembolism alone results in ~300,000 and 550,000 deaths in the US and Europe, respectively, and an even larger number of non-fatal events [1] , [2] . Oral anticoagulants of the 4-hydroxycoumarin (4HC) class are commonly used to treat thromboembolic diseases. Interestingly, the anticoagulant function of 4HC derivatives was initially discovered when livestock fed with mouldy sweet clover forage (called ‘sweet clover disease’) developed fetal animal disease, characterized by internal bleeding. Indeed, fermentation of plant materials containing melilotoside by moulds causes the formation of 4HC and its derivative dicoumarol. The latter demonstrates the blood anticoagulant property by antagonism of vitamin K and acted as a forerunner of the synthetic anticoagulants typified by warfarin [3] . Warfarin is one of the most prescribed oral anticoagulants worldwide and had a global market value of $300 million in 2008 (ref. 4 ). In Europe, acenocoumarol and phenprocoumon are also commonly administered [5] . These drugs share the 4HC core structure but differ in 3-substitution on the pyrone ring and can be chemically synthesized using 4HC as an immediate precursor [6] , [7] . In past decades, various strategies were developed to chemically synthesize 4HC using petro-derived chemicals, such as phenol, acetosalicylate, methylsalicylate or 2′-hydroxyacetophenone as starting materials [8] . Nevertheless, increasing concerns on petroleum depletion and environmental issues have stimulated greater efforts towards the development of biological processes capable of utilizing renewable resources instead of petro-based chemicals. The convergence of genetics, bioinformatics and metabolic engineering greatly promoted the engineered biosynthesis of a variety of pharmaceutically important compounds in heterologous microbial hosts, for example, artemisinic acid [9] , taxadiene [10] , caffeic acid [11] , benzylisoquinoline alkaloids [12] , terpenoids [13] , anthocyanin [14] , flavonoids [15] and resveratrol [16] . The success of these studies was built on a thorough understanding of the products’ native biosynthetic mechanisms, especially genetic and biochemical properties of the involved enzymes. However, lack of knowledge in these aspects hindered the reconstitution of the biosynthesis of pharmaceutically important 4HC. Although it was proposed that 4HC was formed when melilotoside-containing plant materials were fermented by moulds and a biosynthetic scheme was described by isotopic labelling analysis [17] , key enzymes have not yet been identified [18] . Several recent studies revealed that the ortho -hydroxylated cinnamoyl-CoA analogues can form coumarins by spontaneous trans/cis isomerization and lactonization [19] , [20] , [21] , suggesting that the pathway might be shunted from trans -2-coumaroyl-CoA to generate coumarin rather than 4HC. Recently, Liu et al . [22] identified several biphenyl synthases (BISs) from Sorbus aucuparia that catalyse the formation of 3,5-dihydroxybiphenyl through decarboxylative condensation of three malonyl-CoA molecules with benzoyl-CoA. Surprisingly, when ortho -hydroxybenzoyl-CoA (salicoyl-CoA) was used in place of benzoyl-CoA as a substrate, only one molecule of malonyl-CoA was condensed to form 4HC, suggesting that the ortho -hydroxyl group facilitates the intramolecular cyclization without the condensation of another two malonyl-CoA molecules. Accordingly, a biosynthetic pathway extended from plant salicylate biosynthesis was proposed. However, the same study reported that S. aucuparia cells cannot produce 4HC natively even with the presence of supplemented salicylate [22] , indicating the absence of a CoA ligase that can convert salicylate to salicoyl-CoA. In addition, salicylate biosynthesis in plants has not been fully elucidated [23] . In this work, we present the design and constitution of a novel biosynthetic mechanism affording the de novo biosynthesis of 4HC in E. coli . Remarkably, an FabH-like quinolone synthase from Pseudomonas aeruginosa is identified by function-based bioprospecting, which eliminates the bottleneck of the biosynthetic mechanism. Preliminary optimization via metabolic engineering demonstrates its scale-up potential, leading to efficient biosynthesis of 4HC and in situ semisynthesis of warfarin. Retro-design of 4HC biosynthesis 4HC is a direct precursor of natural and synthetic anticoagulants ( Fig. 1 ). Its biosynthesis has not been fully understood as mentioned above ( Fig. 2a ). However, identification of the 4HC-forming reaction catalysed by BIS provided an opportunity to explore the combinatorial biosynthesis of 4HC. The design was first focused on the establishment of a reaction that can provide the substrate salicoyl-CoA for BIS. We speculated that esterification of salicylate with coenzyme A is a reaction that might be catalysed by certain CoA transferase/ligase. By searching the enzyme database (BRENDA) and the literature, we found only a few enzymes with salicylate:CoA ligase (SCL) activity, including SdgA (involved in salicylate degradation in Streptomyces sp. WA46), MdpB2 and SsfL1 (involved in maduropeptin and tetracycline SF2575 biosynthesis in Actinomadura madurae ATCC39144 and Streptomyces sp. SF2575, respectively) [24] , [25] , [26] . Besides, some benzoate:CoA ligases also exhibited weak side activity towards salicylate [27] , [28] . To further achieve de novo biosynthesis of 4HC, a metabolic connection has to be established between salicylate and the host’s metabolism. In nature, salicylate is produced not only by plants as a signal molecule but also by some bacteria as an intermediate in siderophore biosynthesis [29] , [30] . Compared with the intricate plant pathways, bacteria generate salicylate using more straightforward strategies. For instance, in Pseudomonas and Mycobacterium species, salicylate formation requires only two enzymes that are isochorismate synthase (ICS) and isochorismate pyruvate lyase (IPL) by shunting chorismate from the shikimate pathway [29] , [30] . Taken together, a novel biosynthetic mechanism for 4HC is established by grafting the enzymatic reactions catalysed by ICS, IPL, SCL and BIS onto the shikimate pathway ( Fig. 2b ). 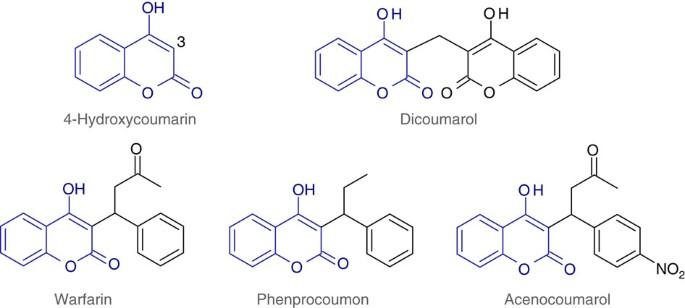Figure 1: Molecular structures of 4HC class anticoagulants. Dicoumarol is a natural 4HC derivative and served as the earliest anticoagulant; whereas warfarin, phenprocoumon and acenocoumarol are the most widely prescribed synthetic 4HC anticoagulants. These compounds share the 4HC core structure but differ in substitution at 3-position on the pyrone ring. Figure 1: Molecular structures of 4HC class anticoagulants. Dicoumarol is a natural 4HC derivative and served as the earliest anticoagulant; whereas warfarin, phenprocoumon and acenocoumarol are the most widely prescribed synthetic 4HC anticoagulants. These compounds share the 4HC core structure but differ in substitution at 3-position on the pyrone ring. 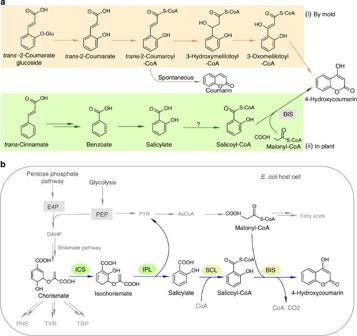Figure 2: Schematic representations of natural and artificial 4HC biosynthetic pathways. (a) Previously proposed natural 4HC biosynthetic routes. Scheme i in the yellow box describes the mould-mediated 4HC biosynthesis; scheme ii in the blue box represents a proposed microbe-independent pathway in plant. Question mark indicates a questionable catalytic step that was not identified. (b) The artificial 4HC biosynthetic mechanism designed in this study. Blue-coloured arrows indicate non-native catalytic steps; gray-coloured arrows indicate theE. coliendogenous metabolism. Critical enzymes ICS and IPL, and SCL and BIS are highlighted with green- and yellow-coloured circles, respectively, representing upper and lower modules. E4P:D-erythrose-4-phosphate; PEP: phosphoenolpyruvate; PYR: pyruvate; AcCoA: acetyl-CoA. Full size image Figure 2: Schematic representations of natural and artificial 4HC biosynthetic pathways. ( a ) Previously proposed natural 4HC biosynthetic routes. Scheme i in the yellow box describes the mould-mediated 4HC biosynthesis; scheme ii in the blue box represents a proposed microbe-independent pathway in plant. Question mark indicates a questionable catalytic step that was not identified. ( b ) The artificial 4HC biosynthetic mechanism designed in this study. Blue-coloured arrows indicate non-native catalytic steps; gray-coloured arrows indicate the E. coli endogenous metabolism. Critical enzymes ICS and IPL, and SCL and BIS are highlighted with green- and yellow-coloured circles, respectively, representing upper and lower modules. E4P: D -erythrose-4-phosphate; PEP: phosphoenolpyruvate; PYR: pyruvate; AcCoA: acetyl-CoA. Full size image Conversion of salicylate to 4HC Conversion of salicylate to 4HC (the lower module) by SCL and BIS is a non-natural pathway and the centrepiece of this design. The three identified BISs were reported to show different preferences towards salicoyl-CoA; BIS3 was selected for pathway construction due to its higher k cat value [22] . To obtain an optimal SCL, we measured the catalytic parameters of SdgA and MdpB2 after evaluating all the reported SCLs. The enzyme assays revealed that SdgA ( K m =4.05 μM, k cat =10.63 s −1 ) possesses about 2-fold higher substrate affinity and 10-fold higher activity than MdpB2 ( K m =8.53 μM, k cat =1.18 s −1 ) ( Supplementary Fig. S1 and Supplementary Table S1 ). To further test their biosynthetic potential in vivo , an expression vector (pZE-BIS3-SdgA) carrying the genes of BIS3 and SdgA was constructed and introduced into E. coli . The strain was cultured in the presence of 1 mM salicylate for 24 h. High-performance liquid chromatography (HPLC) analysis showed that the strain produced 2.3±0.2 mg l −1 of 4HC with ~3–6 mg l −1 salicylate consumed ( Supplementary Fig. S2 ). Biosynthesis of salicylate We borrowed the biosynthetic strategy from Pseudomonas involving ICS and IPL to establish the salicylate biosynthesis (the upper module) in E. coli . First, to screen for a potent ICS, the enzymes PchA (from P. aeruginosa ), EntC and MenF (from E. coli ) were overexpressed and purified for enzyme kinetic studies. The enzyme assays indicated that EntC ( K m =11.93 μM and k cat =2.12 s −1 ) is much more active than MenF ( K m =6.75 μM and k cat =0.13 s −1 ) and PchA ( K m =3.69 μM and k cat =0.20 s −1 ) ( Supplementary Fig. S3 and Supplementary Table S1 ). Then the activity of IPLs from Pseudomonas fluorescence and P. aeruginosa was estimated by coupled enzyme assays as the substrate isochorismate is neither commercially available nor chemically stable. The results showed that the former enzyme (PfPchB, estimated turnover number=15.8 s −1 ) is slightly more active than the latter one (PaPchB, estimated turnover number=11.2 s −1 ). Therefore, EntC and PfPchB were selected for the test of salicylate biosynthesis in vivo . We consecutively cloned the genes of EntC and PfPchB into the vector pZE12-luc as an operon, generating pZE-EP. As we expected, the E. coli strain harbouring pZE-EP obtained the capability of producing salicylate. By the end of 32 h, 158.5±2.5 mg l −1 of salicylate was accumulated in the cultures following a growth-dependent production pattern ( Supplementary Fig. S4 ). Validation and diagnosis of the 4HC biosynthetic mechanism With the validated upper and lower modules, further efforts were directed to the validation of the complete 4HC biosynthetic mechanism. The genes encoding EntC, PfPchB, BIS3 and SdgA were consecutively cloned into the vector pZE12-luc as an operon, generating a plasmid pZE-EPBS. However, the E. coli strain harbouring pZE-EPBS only produced a trace amount of 4HC (<0.2 mg l −1 ) but accumulated a large amount of salicylate (156.2±18.7 mg l −1 ) after 48 h production in shake flasks. The result suggested that the upper module performed well in the full pathway; whereas the bottleneck lay in the lower module. To locate the rate-limiting step, we designed and performed an in vitro complementation assay in which excess amounts of purified SdgA and/or BIS3 were supplemented into the crude extract of the E. coli cells expressing the full pathway. As shown in Fig. 3 , without supplemented enzymes, the crude extract can only convert salicylate to 4HC at a very low rate (0.18 mg l −1 h −1 ) in the presence of required cofactors; whereas the presence of purified SdgA and BIS3 significantly improved the rate (8.82 mg l −1 h −1 ), indicating that the purified enzymes functioned well in this assay system (positive control). When purified SdgA was supplemented alone into the crude extract, the conversion rate was not obviously increased (0.24 mg l −1 h −1 ). Noticeably, when purified BIS3 was added alone, the 4HC formation was recovered to a rate (7.83 mg l −1 h −1 ) comparable with that of the positive control, indicating that BIS3 was a major bottleneck in the pathway. We speculated that the low in vivo activity of BIS3 might result from the slow kinetics, suboptimal expression, instability or cross-species incompatibility issues. To overcome this bottleneck, searching for a superior substitute was our first choice. 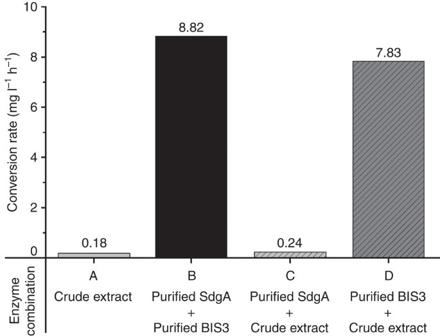Figure 3:In vitrocomplementation assay for examining the rate-limiting enzyme. Four combinations of enzymes were tested forin vitro4HC formation. Crude extract was prepared from the lysed cells of theE. colistrain expressing the full pathway (E. coli/pZE-EPBS). Figure 3: In vitro complementation assay for examining the rate-limiting enzyme. Four combinations of enzymes were tested for in vitro 4HC formation. Crude extract was prepared from the lysed cells of the E. coli strain expressing the full pathway ( E. coli /pZE-EPBS). Full size image Bioprospecting for a superior substitute to BIS BIS is a subclass of chalcone synthase (CHS)-like type III polyketide synthases (PKSs). However, no other type III PKS with sequence similarity has been identified to catalyse the 4HC-forming reaction. By structure-based examination of bacterial secondary metabolites, we identified that 4-hydroxy-2(1H)-quinolone in P. aeruginosa shares high structural similarity with 4HC [31] . The formation of 4-hydroxy-2(1H)-quinolone is catalysed by a β-ketoacyl-ACP synthase III (FabH)-type quinolone synthase (PqsD) via decarboxylative condensation of malonyl-CoA or -ACP with anthraniloyl-CoA and spontaneous intramolecular cyclization [31] , [32] . Despite having a tautomer 2,4-dihydroxyquinoline, 4-hydroxy-2(1H)-quinolone is the predominant form at physiological pH [33] ( Fig. 4b ). Considering the high similarity in substrate and product structures and catalytic mechanisms between the two reactions, we reasoned that PqsD may also accept salicoyl-CoA as a substrate to form 4HC, as BIS does ( Fig. 4a ). To test this hypothesis, we replaced the BIS3 gene with PqsD coding sequence in the lower module, generating the plasmid pZE-PqsD-SdgA (pZE-PS). The E. coli strain carrying pZE-PS completely converted 2 mM of salicylate (276 mg l −1 ) into 4HC within ~7 h with a yield of over 99%, indicating the high activity of PqsD towards salicoyl-CoA. The produced 4HC has identical HPLC retention time and ultraviolet absorption profile with its commercial standard. Its identity was further confirmed by electron spray ionization-mass spectroscopy (ESI-MS) and NMR analysis ( Supplementary Figs S5-S8 and Supplementary Table S2 ). 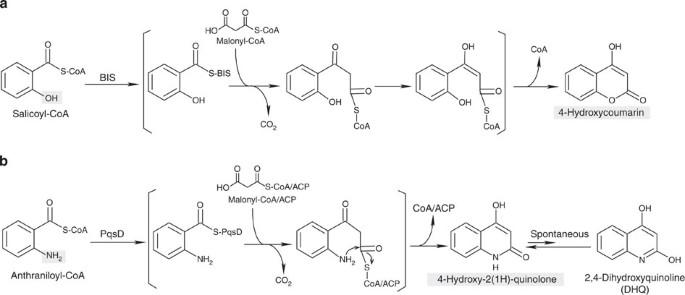Figure 4: Comparison of the reaction mechanisms of biphenyl synthase and Pseudomonas quinolone synthase. Biphenyl synthase catalyses the decarboxylative condensation of malonyl-CoA with salicoyl-CoA, after which intramolecular cyclization takes place to form 4HC. Pseudomonas quinolone synthase was reported to condense malonyl-CoA/malonyl-ACP and anthraniloyl-CoA. Then similar intramolecular cyclization takes place to form 4-hydroxy-2(1H)-quinolone, which is spontaneously interchangeable to its tautomer 2,4-dihydroxyquinoline (DHQ). Under physiological conditions 4-hydroxy-2(1H)-quinolone is the dominant form. Figure 4: Comparison of the reaction mechanisms of biphenyl synthase and Pseudomonas quinolone synthase. Biphenyl synthase catalyses the decarboxylative condensation of malonyl-CoA with salicoyl-CoA, after which intramolecular cyclization takes place to form 4HC. Pseudomonas quinolone synthase was reported to condense malonyl-CoA/malonyl-ACP and anthraniloyl-CoA. Then similar intramolecular cyclization takes place to form 4-hydroxy-2(1H)-quinolone, which is spontaneously interchangeable to its tautomer 2,4-dihydroxyquinoline (DHQ). Under physiological conditions 4-hydroxy-2(1H)-quinolone is the dominant form. Full size image Metabolic engineering for improved 4HC biosynthesis We first reconstituted the improved biosynthetic mechanism in E. coli by introducing the two modules as dual operons using the high-copy plasmid pZE-EP-PS. The E. coli strain carrying pZE-EP-PS (Strain A, Fig. 5a ) produced 42.3 mg l −1 of 4HC without addition of any intermediates. Meanwhile, a trace amount of salicylate was detected in the cultures, indicating that the lower module functioned well with this expression strategy and almost completely converted endogenous salicylate to 4HC. However, this expression strategy decreased the efficiency of the upper module. According to the stoichiometry, 42.3 mg l −1 of 4HC should be generated from 36.1 mg l −1 salicylate, which is much less than the production obtained with the E. coli strain only expressing the upper module (pZE-EP). We speculated that the decrease in salicylate-producing capability might be attributed to the following two reasons. First, the two adjacent operons on the same plasmid might interfere with each other and second, the incongruous expression of the upper and lower modules may have caused metabolic imbalance. To test this hypothesis, we coexpressed the lower module operon (PqsD-SdgA) using a medium-copy plasmid (pCS-PS) together with pZE-EP in E. coli (Strain B, Fig. 5b ). Strain B produced 108.9 mg l −1 4HC in 18 h with no measurable salicylate accumulated. Furthermore, we explored the performance of another construct pZE-EPPS in which the genes encoding the full pathway enzymes were consecutively cloned as one operon. E. coli harbouring pZE-EPPS (Strain C, Fig. 5c ) produced 207.7 mg l −1 4HC in 24 h with 21.6 mg l −1 salicylate left unconverted. With this expression strategy, the production of 4HC was improved by fivefold compared with the initial construct, suggesting that gene organization and operon configuration have a great impact on the biosynthetic capability of heterologous pathways. 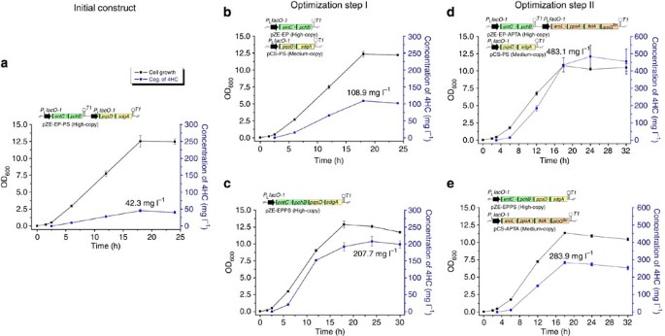Figure 5: Growth and production profiles of the constructed 4HC-producingE. colistrains. (a) Strain A (E. colicarrying pZE-EP-PS) expresses the upper module (EP) and lower module (PS) with two operons on the high-copy plasmid; panelsbandcindicate the modular optimization by adjusting gene organization, copy number and operon configuration. Strain B separately expresses upper module (EP) and lower module (PS) on the high-copy and the medium-copy plasmids, respectively, whereas Strain C expresses the full pathway within the same operon on the high-copy plasmid; panelsdandeindicate improving precursor availability by overexpressingaroL,ppsA,tktAandaroGfbr(APTA) on the high-copy and medium-copy plasmids, respectively. Characteristics of the plasmid(s) carried byE. coliare shown on the upper-left corner of each graph. All data are reported as mean±s.d. from three independent experiments (n=3). Error bars are defined as s.d. Figure 5: Growth and production profiles of the constructed 4HC-producing E. coli strains. ( a ) Strain A ( E. coli carrying pZE-EP-PS) expresses the upper module (EP) and lower module (PS) with two operons on the high-copy plasmid; panels b and c indicate the modular optimization by adjusting gene organization, copy number and operon configuration. Strain B separately expresses upper module (EP) and lower module (PS) on the high-copy and the medium-copy plasmids, respectively, whereas Strain C expresses the full pathway within the same operon on the high-copy plasmid; panels d and e indicate improving precursor availability by overexpressing aroL , ppsA , tktA and aroG fbr (APTA) on the high-copy and medium-copy plasmids, respectively. Characteristics of the plasmid(s) carried by E. coli are shown on the upper-left corner of each graph. All data are reported as mean±s.d. from three independent experiments ( n =3). Error bars are defined as s.d. Full size image We further speculated that boosting the availability of chorismate and malonyl-CoA, the two major intermediates of 4HC biosynthesis, may divert more metabolic flux towards product formation. Chorismate is a critical intermediate in the shikimate pathway, of which the rate-limiting steps have been identified and the regulation mechanism has been well studied. As shown in Supplementary Fig. S9 , the 3-deoxy- D -arabino-heptulosonate-7-phosphate synthases in E. coli encoded by aroG , aroF and aroH are feedback-inhibited by phenylalanine, tyrosine and tryptophan, respectively [34] . Moreover, the erythrose-4-phosphate and phosphoenolpyruvate availability limit can be alleviated by overexpressing transketolase (encoded by tktA ) and phosphoenolpyruvate synthase (encoded by ppsA ), respectively [35] . Besides, shikimate kinase (encoded by aroK / aroL ) was proved to be another bottleneck, which can be eliminated by the overexpression of aroL [36] . Based on this knowledge, we cloned aroL , ppsA , tktA and the feedback-inhibition-resistant aroG ( aroG fbr ) into pCS27 generating a chorismate-boosting plasmid pCS-APTA. The E. coli strain carrying pZE-EPPS and pCS-APTA (Strain E, Fig. 5e ) produced 283.9 mg l −1 4HC in 18 h, a 37% increase compared with its parent Strain C. Meanwhile, we created another construct by inserting the P L lacO1-APTA operon into pZE-EP generating a dual-operon plasmid pZE-EP-APTA, which was cotransferred together with pCS-PS into E. coli (Strain D, Fig. 5d ). Remarkably, Strain D produced 483.1 mg l −1 4HC in 24 h, reflecting 4.4- and 11.4-fold increases compared with its parent (Strain B) and Strain A, respectively. Meanwhile, we detected the accumulation of salicylate at the concentrations of 197.6 and 222.3 mg l −1 at 24 h for Strains D and E, respectively, due to the boosting of the shikimate pathway. Furthermore, we examined the impact of malonyl-CoA on the production of 4HC. As it has been reported that overexpression of acetyl-CoA carboxylase ( accABCD ) and biotin ligase ( birA ) can increase the availability of malonyl-CoA [37] , [38] , we cloned genes accADBC and birA into pSA74 generating a malonyl-CoA-enhancing plasmid pSA-ACCB. The introduction of pSA-ACCB into Strain E led to slightly improved production of 4HC (313.4 mg l −1 , 11% higher than Strain E). However, the pSA-ACCB exerted a negative influence on Strain D ( E. coli /pZE-EP-APTA and pCS-PS), manifesting a dramatic fall in the 4HC production (184.1 mg l −1 ). The results indicated that: (1) malonyl-CoA availability might not be a dominant limiting factor in 4HC production; (2) the overexpression of accADBC and birA could improve malonyl-CoA availability but might cause metabolic burden in strain D, which offset their benefit in boosting malonyl-CoA availability. Semisynthesis of warfarin With tentative optimization, the resulting E. coli strain demonstrated great scale-up potential for 4HC production. Then we explored the feasibility of in situ semisynthesis of warfarin via a green chemistry approach [39] . To this end, the other precursor benzyldeneacetone and the catalyst ( S,S )-1,2-diphenylethylenediamine were added into the supernatant of the strain D culture (containing about 500 mg l −1 4HC) and incubated in a sonication bath for 3 h. Quantitative HPLC analysis indicated that 43.7±2.6 mg l −1 warfarin was generated in the supernatant corresponding to a molar yield of 4.6% ( Supplementary Fig. S10 ). The low yield might be due to the facts that: (1) the aqueous condition is not optimal for the Michael addition reaction; (2) the 4HC concentration is lower than the optimal concentration for warfarin synthesis. Recent advances of metabolic engineering have allowed the microorganisms to be engineered to enable the efficient and environmental-friendly production of valuable molecules. Although the design principles for constituting a productive pathway are explored and yet to be well-established, recruitment of catalytically superior and host-suitable enzymes should be the primary one in the principles, which is evidenced by this work and previous studies [40] , [41] , [42] . Conventionally, sequence-based bioprospecting aided by bioinformatics and computational tools is an effective approach in searching for such candidates. For instance, BLAST search using the sequence information of an enzyme with known function as a query may be employed to identify homologous enzymes from various organisms capable of catalysing the same type of reaction but exhibiting enhanced activity and desired substrate specificity [43] . In our work, we first developed an in vitro complementation assay to accurately locate the rate-limiting step in the 4HC biosynthesis. To eliminate the bottleneck, we further employed a function-based bioprospecting strategy to search for a more suitable enzyme. We successfully identified 4-hydroxy-2(1H)-quinolone synthase for efficient microbial biosynthesis of 4HC totally based on the similarity in catalytic mechanisms and substrate/product structures between BIS and 4-hydroxy-2(1H)-quinolone synthase. Indeed, 4-hydroxy-2(1H)-quinolone synthase shares low sequence identity with BIS (~25%) but exhibits functional and catalytic attributes of both CHS and FabH-like enzymes. On one hand, it can catalyse the condensation of malonyl-CoA as well as intramolecular cyclization, which are the properties of CHS-like PKS; on the other hand, it can also condense malonyl-ACP in a manner of FabH [32] . So far, the function-based bioprospecting can only be performed manually by analysing and comparing enzyme catalytic mechanisms. However, we envision the development of computational tools that can effectively predict the catalytic substitutability of enzymes with low sequence correlation will further enhance our capability of engineering combinatorial biosynthesis. With efficient enzymes available for each catalytic step, optimization of the pathway by adjusting expression level of individual enzymes is also critical for the pathway’s overall performance. First, inharmonious expression of pathway enzymes may waste cellular resources for the formation of unnecessary RNAs, proteins or intermediates. Besides, overexpression of some exotic enzymes is stressful or toxic to host cells, which may result in growth retardation and undesired adaptive responses, hence reducing yield and productivity [44] . Methodologies have been developed to determine the ideal expression level and have been successfully applied by fine-tuning the expression level of pathway enzymes and modules, such as the use of plasmids with different copy numbers, promoters with various transcription strengths and synthetic RBSs with different translation efficiencies [10] , [45] , [46] , [47] . In our case, modular optimization by adjusting gene organization, copy number and operon configuration also led to a ~fivefold increase in the 4HC titre (Strain C versus Strain A). In conclusion, this work achieves microbial production of the pharmaceutically important drug precursor 4HC for the first time and demonstrates great scale-up potential. The findings provide a new insight into the non-natural 4HC biosynthesis, which can serve as a starting point for expanding the molecular diversity of coumarin compounds through synthetic chemistry and biology approaches. Experimental materials Plasmids were generated via either regular cloning or Gibson assembly ( Supplementary Methods ) [48] . The E. coli strain XL1-Blue was used for plasmid propagation and gene cloning; BL21 star (DE3) was used for recombinant protein expression and purification; BW25113 containing F’ from XL1-Blue was used as the host strain for the biosynthesis of salicylate and 4HC. The characteristics of all the strains and plasmids used in this study are described in Supplementary Table S3 . Luria-Bertani (LB) medium was used to grow E. coli cells for plasmid construction, propagation and inoculum preparation. The biosynthesis medium M9Y contains (per liter): glycerol (20 g), yeast extract (5 g), NH 4 Cl (1 g), Na 2 HPO 4 (6 g), KH 2 PO 4 (3 g), NaCl (0.5 g), MgSO 4 ·7H 2 O (2 mmol), CaCl 2 ·2H 2 O (0.1 mmol) and vitamin B1 (1.0 mg). In all, 100 μg ml −1 of ampicillin, 50 μg ml −1 of kanamycin and/or 30 μg ml −1 of chloramphenicol were added when necessary. Enzyme assays of SCLs To evaluate the activity of SCLs (SdgA and MdpB2), the E. coli strain BL21 Star (DE3) was transformed with pET-SdgA and pET-MdpB2 separately. The obtained transformants were preinoculated in LB medium containing 100 μg ml −1 of ampicillin and grown aerobically at 37°C overnight. Next day, the preinoculums were transferred into 50 ml of fresh LB medium at a volume ratio of 1:100. The cultures were left to grow at 37°C till the OD 600 values reached 0.6–0.8 and were then induced with 1.0 mM isopropyl-β-D-thiogalactoside (IPTG). Protein expression was conducted at 30°C for another 5 h. The cells were harvested and the proteins were purified with the His-Spin Protein Miniprep kit (ZYMO RESEARCH). The BCA kit (Pierce Chemicals) was used to estimate protein concentrations. The SCL enzyme assays were performed according to the method described by Ishiyama et al . [24] with modifications. The 1 ml reaction system contained 785 μl of Tris-HCl (pH=7.5, 100 mM), 5 μl of the purified enzyme (SdgA or MdpB2), 10 μl of MgCl 2 (0.5 M), 50 μl of ATP (100 mM), 50 μl of coenzyme A (5 mM), 100 μl of salicylate (100 μM, 200 μM, 500 μM and 1 mM). The reactions lasted 0.5 min for SdgA and 2.5 min for MdpB2, respectively, and then were terminated by acidification with 20 μl of HCl (20%). The reaction rates were calculated according to the salicylate consumption at 30°C, which was measured by HPLC. Enzyme assays of ICSs The kinetic parameters of the ICSs: EntC, MenF and PchA were determined using coupled assays [49] . IPL from P. aeruginosa (PaPchB) was used to convert isochorismate to salicylate, which was quantified by HPLC. The 1 ml reaction system contained 866 μl of Tris-HCl (pH=7.5, 100 mM), 20 μl of MgCl 2 (0.5 M), 0.1 μM of purified ICS (EntC, MenF or PchA), 0.5 μM of purified PaPchB, 100 μl of chorismic acid (100 μM, 200 μM, 500 μM and 1 mM). The reactions lasted 1 min for EntC and 5 min for MenF and PchA, respectively, and then were terminated by acidification with 20 μl of HCl (20%). The reaction rates were calculated according to the salicylate accumulation at 30°C. The kinetic parameters were estimated by using OriginPro8 through non-linear regression of the Michaelis–Menten equation. Coupled enzyme assays for IPLs First, purified enzyme EntC was used to convert an excess amount of chorismic acid into IPL’s substrate isochorismate. The 1 ml reaction system containing Tris-HCl (100 mM, pH=7.5), MgCl 2 (5 mM), purified EntC (0.5 μM), chorismic acid (100 μM) was incubated at 30°C for 30 min. Then the purified PaPchB or PfPchB was added into the reaction system and incubated for 30 s after which the reactions were terminated by acidification with 20 μl of HCl (20%). The enzyme turnover numbers were estimated according to the generation of salicylate, which was measured by HPLC. Feeding experiments Feeding experiments were conducted to examine the conversion of salicylate to 4HC. The E. coli strain carrying pZE-BIS3-SdgA or pZE-PS was inoculated in 3 ml LB medium and grown overnight at 37°C. Subsequently, 200 μl overnight cultures were re-inoculated into 20 ml of M9Y medium and grown at 37°C with shaking (250 r.p.m.). The expression of the enzymes was induced by adding IPTG to a final concentration of 0.5 mM when the OD 600 values reached 0.6–0.7. At the same time, 1 mM of salicylate was added into the cultures and the cultures were shaken at 30°C for several hours, which was followed by HPLC analysis. De novo biosynthesis of salicylate and 4HC Overnight cultures (100 μl) of salicylate or 4HC-producing strains were inoculated into M9Y medium (10 ml) containing appropriate antibiotics and cultivated at 37 °C with shaking at 300 r.p.m. When the OD 600 values of the cultures reached ~0.6, IPTG was added to the cultures to a final concentration of 0.5 mM. Then the cultures were transferred to 30°C for salicylate and 4HC biosynthesis. Samples were taken every other hour and analysed by HPLC. In vitro complementation assay The E. coli strain carrying the plasmid pZE-EPBS was preinoculated into 3 ml LB liquid medium containing 100 μg ml −1 of ampicillin and grown at 37°C overnight with shaking at 300 r.p.m. The following day, 1 ml of the preinoculum was added to 50 ml of fresh M9Y medium. The culture was left to grow at 37°C till the OD 600 value reached ~0.6 and then induced with 0.5 mM IPTG. The expression of the pathway enzymes was conducted at 30°C for another 5 h. The cells were harvested and re-suspended in 2 ml of Tris-HCl buffer (100 mM, pH=7.5) and then lysed by French Press. The soluble fraction was collected by ultracentrifugation and used as the crude enzyme extract for the complementation assay. The 1 ml reaction system first contained Tris-HCl (100 mM, pH=7.5), MgCl 2 (5 mM), ATP (5 mM), coenzyme A (0.25 mM), salicylate (0.2 mM) and crude extract (50 μl) with/without purified SdgA (20 μl). After 30 min reaction, 100 μl of malonyl-CoA (2 mM) and 50 μl of crude extract with/without purified BIS3 (20 μl) were supplemented into the reaction system. The reactions were finally terminated in another 0.5–2 h by acidification. The reaction rates were calculated according to the generation of 4HC that was measured by HPLC. The protein concentrations of purified BIS3 and SdgA were 1,200 and 395 mg l −1 , respectively. Semi-synthesis of warfarin The culture containing ~500 mg l −1 of produced 4HC was centrifuged to remove the cells. Then 1 g l −1 of benzyldeneacetone and 100 mg l −1 of catalyst ( S,S )-1,2-diphenylethylenediamine were added into the supernatant followed by incubation in the sonication bath for 3 h. The production of warfarin was analysed by HPLC. HPLC quantitative analysis 4-Hydroxycoumarin (from ACROS ORGANICS), salicylate (from ACROS ORGANICS) and warfarin (from MP Biomedicals) were purchased as the standards. Both the standards and samples were quantitatively analysed by HPLC (Dionex Ultimate 3000) with a reverse-phase ZORBAX SB-C18 column and an Ultimate 3000 Photodiode Array Detector. Solvent A was sodium acetate solution (20 mM, pH=5.5) and solvent B was 100% methanol. The following gradient was used for 4HC and salicylate analysis at a flow rate of 1 ml min −1 : 5–50% solvent B for 15 min, 50–5% solvent B for 1 min and 5% solvent B for an additional 4 min. For warfarin analysis, the gradient was from 20 to 80% solvent B. Quantification was based on the peak areas referring to the commercial standards at the wavelength of 285 nm. Samples containing over 200 mg l −1 of products were diluted before running HPLC to maintain a linear concentration–peak area relationship. ESI-MS and NMR analysis For ESI-MS analysis, the peak corresponding to 4HC was collected from HPLC, extracted with acetyl acetate and dissolved in H 2 O. ESI-MS analysis was conducted using the Perkin Elmer Sciex API I plus mass spectrometer. For NMR analysis, the biosynthesized 4HC was extracted from the culture with the same volume of acetyl acetate. Then the extract was dried by a vacuum evaporator, dissolved with dimethylsulphoxide (DMSO) and diluted with water. Further purification was performed by collecting the 4HC fraction from HPLC. The collected fraction was extracted again with acetyl acetate, dried and re-dissolved in DMSO. Then the purified 4HC (roughly 0.2–0.3 mg in ~50 μl DMSO) was diluted in 600 μl DMSO- d6 . The NMR analysis was conducted using 500-MHz Varian Unity Inova with a 5-mm Broad Band Detection Probe at 25°C. The solvent DMSO was used as the reference compound. 1 H, 13 C and gHSQC (gradient heteronuclear single quantum coherence) analysis were conducted ( Supplementary Fig. S6-S8 ). The carbons and protons were assigned by referring to the data from Spectral Database for Organic Compounds (SDBS No. : 6281) ( Supplementary Fig. S11 ). How to cite this article: Lin, Y. et al . Microbial biosynthesis of the anticoagulant precursor 4-hydroxycoumarin. Nat. Commun. 4:2603 doi: 10.1038/ncomms3603 (2013).